Silicon carbide-derived carbon nanocomposite as a substitute for mercury in the catalytic hydrochlorination of acetylene Acetylene hydrochlorination is an important coal-based technology for the industrial production of vinyl chloride, however it is plagued by the toxicity of the mercury chloride catalyst. Therefore extensive efforts have been made to explore alternative catalysts with various metals. Here we report that a nanocomposite of nitrogen-doped carbon derived from silicon carbide activates acetylene directly for hydrochlorination in the absence of additional metal species. The catalyst delivers stable performance during a 150 hour test with acetylene conversion reaching 80% and vinyl chloride selectivity over 98% at 200 °C. Experimental studies and theoretical simulations reveal that the carbon atoms bonded with pyrrolic nitrogen atoms are the active sites. This proof-of-concept study demonstrates that such a nanocomposite is a potential substitute for mercury while further work is still necessary to bring this to the industrial stage. Furthermore, the finding also provides guidance for design of carbon-based catalysts for activation of other alkynes. Polyvinylchloride is one of the most widely used plastics in different areas of human life. In developing countries with rich coal reserves, vinyl chloride (the monomer of polyvinylchloride) is primarily manufactured from acetylene via hydrochlorination, which uses mercuric chloride (HgCl 2 ) supported on activated carbon (AC) as the catalyst. However, HgCl 2 is apt to be reduced by acetylene and sublimates during reaction. This not only leads to deactivation of the catalyst, but also contaminates the product, and may cause severe environmental problems and threats to human health [1] . Recently, more than 140 countries accepted ‘The Minamata Convention on Mercury’ and promised to reduce and eventually eliminate mercury pollution by 2020 (ref. 2 ). Furthermore, the ready sublimation of mercury also restricts the hydrochlorination space velocity (30–50 h −1 ) and reaction temperature (130–180 °C), and hence limits the production capacity. In addition, AC is easily crushed under reaction conditions, resulting in further loss of the active mercuric species and eventual deactivation of the catalyst. Therefore, efforts are ongoing to replace the harmful and scarce mercury as well as the carbon support [3] , [4] , [5] , [6] , [7] , [8] , [9] , [10] , [11] , however AC-supported HgCl 2 remains the catalyst for industrial hydrochlorination of acetylene to date. The pioneering work and systematic studies carried out by Hutchings and coworkers on more than 30 metal chlorides showed that AuCl 3 may be the best replacement of HgCl 2 for this process because of its high activity [5] , [6] , [7] . Thus, extensive work has been carried out to improve the stability of Au 3+ , for example, by adding a second metal component [6] , [8] , [9] , because Au 3+ is readily reduced to Au 0 under reaction conditions and consequently loses its activity [10] , [11] . Considering the high price and limited reserves of noble metals, exploration of further alternatives particularly with crust-richer elements and even metal-free catalysts remains to be highly imperative. We report in this proof-of-concept study that pyrollic N-doped carbon (N–C) can activate acetylene and hence catalyze the hydrochlorination of acetylene. We synthesize a nanocomposite by growing a N–C layer out of the preshaped silicon carbide (SiC) granules, designated as SiC@N–C. This circumvents the difficulty of shaping nanostructured carbon while yielding a material with good mechanical strength, heat conductivity and chemical stability. The resulting catalyst exhibits a rather high activity and selectivity, and is a potential substitute for toxic mercury in this process. Synthesis and catalytic activity of SiC@N–C Unique catalytic properties of nanostructured-carbon materials have been extensively demonstrated for a wide range of reactions. However, their limitations for practical applications are also recognized such as being difficult to shape and low-mechanical strength. In this respect, SiC may provide a solution by serving as a support for nanostructured carbon [12] , which could combine the merits of both SiC and C. We showed that by reacting SiC with CCl 4 at elevated temperatures, surface silicon atoms can be removed and the remaining carbon atoms reorganize themselves forming small graphene flakes stacking on the SiC surface, as schematically depicted in Fig. 1 . Furthermore, nitrogen can be incorporated in-situ into the sp [2] hybridized network in the presence of NH 3 at 800–1,000 °C. Depending on the reaction conditions (atmosphere, particularly the ratio of NH 3 /CCl 4 , temperature and duration), the textural structure and chemical composition of the carbon layer can be finely modulated while the macro-morphology of the original SiC granules is retained ( Supplementary Fig. 1a ) [12] . The high resolution transmission electron microscopy (HRTEM) images in Fig. 2a and Supplementary Fig. 1b clearly demonstrate a core-shell-like morphology. The SiC core is covered by an amorphous carbon layer, on which few-layer-graphene sheets stack and orient in different directions. The thickness of the carbon layer is usually around 5–8 nm and it is bonded with the underneath SiC. Such an integrated catalyst is expected to provide extra stability against peeling-off with respect to those with carbon layers deposited additionally on top of the substrate. Furthermore, this synthesis method is applicable to commercial polycrystalline SiC granules in different shapes, which is essential for practical applications. 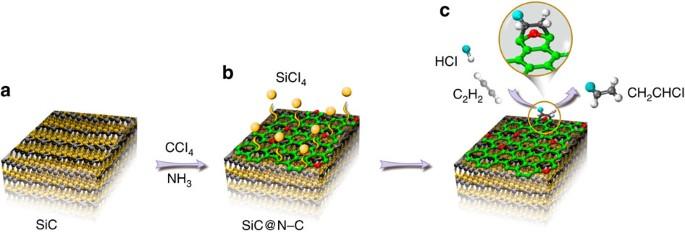Figure 1: Schematic for synthesis of SiC@N-C nanocomposite. (a) SiC granule. (b) SiC@N-C, which is characterized by a layer of N–C grown directly out of and bonded with the SiC substrate under the atmosphere of CCl4and NH3. (c) catalytic conversion of acetylene to vinyl chloride over SiC@N-C. Figure 1: Schematic for synthesis of SiC@N-C nanocomposite. ( a ) SiC granule. ( b ) SiC@N-C, which is characterized by a layer of N–C grown directly out of and bonded with the SiC substrate under the atmosphere of CCl 4 and NH 3 . 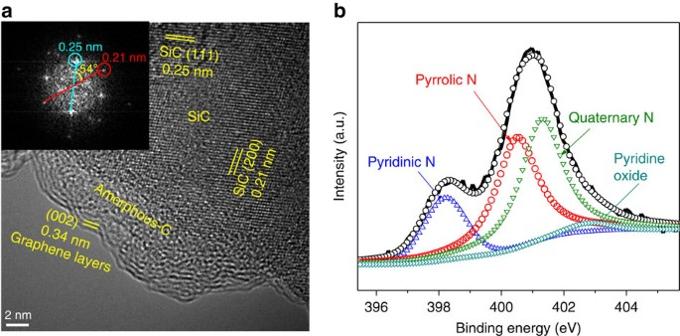Figure 2: Features of SiC@N-C catalyst. (a) HRTEM image of SiC@N-C showing a core-shell-like morphology (scale bar, 2 nm). (b) XPS N1s spectrum for the SiC@N-C catalyst with a total N content of 7.1%. ( c ) catalytic conversion of acetylene to vinyl chloride over SiC@N-C. Full size image Figure 2: Features of SiC@N-C catalyst. ( a ) HRTEM image of SiC@N-C showing a core-shell-like morphology (scale bar, 2 nm). ( b ) XPS N1s spectrum for the SiC@N-C catalyst with a total N content of 7.1%. Full size image Doping carbon with heteroatoms has been demonstrated to be an effective approach to tune its catalytic activities [13] , [14] , [15] , [16] . For example, replacing C with N atoms in graphene layers (so called quaternary N) leads to an increased electron density of states near the Fermi level and the resulting materials can electrocatalyze oxygen reduction reaction without metal species [13] . Introduction of pyridinic-type N species into the carbon network adds basicity [17] , and the derived carbon can be used as a solid-base catalyst [18] . We wondered if such doping of carbon materials can also enhance the adsorption of HCl and activate acetylene, and hence the hydrochlorination of acetylene. 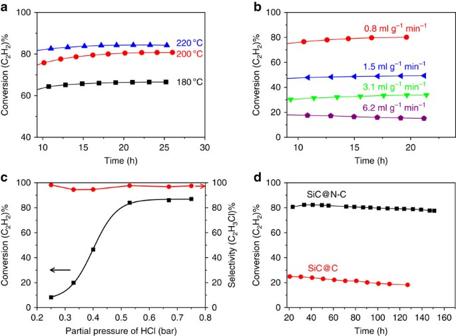Figure 3: Catalytic activity of SiC@N-C. (a) As a function of reaction temperatures. (b) As a function of space velocities. (c) At a varying partial pressure of HCl in the feed stream. (d) Long-term stability test of SiC@N-C. Reactions were carried out at 200 °C, atmospheric pressure, a space velocity of 0.8 ml g−1min−1, HCl/C2H2=1.15/1 (volume ratio) unless otherwise stated. The selectivity to vinyl chloride is above 98%. Figure 3a shows that a SiC@N–C catalyst containing 7.1% N (estimated from X-ray photoelectron spectroscopy (XPS) analysis, Fig. 2b ) gives an acetylene conversion as high as 80% at 200 °C, atmospheric pressure and 0.8 ml g −1 min −1 corresponding to a space velocity of 30 h −1 based on the catalyst volume. In contrast to mercuric chloride which is prone to sublimation under this reaction condition, this catalyst is rather robust. It can be operated at an even higher temperature and space velocity, as shown in Fig. 3a and b , respectively. For example, at 220 °C and 0.8 ml g −1 min −1 the conversion of acetylene reaches 85% and the selectivity to acetylene chloride remains above 98%. Figure 3c indicates that the activity of SiC@N–C is sensitive to the partial pressure of HCl in the feeding stream. The acetylene conversion increases with the partial pressure of HCl and then starts to level off around 0.54 bar, corresponding to HCl/C 2 H 2 =1.15/1 (volume ratio). This is a typical behaviour for the Eley–Rideal (ER) mechanism, suggesting that the reaction proceeds with gas phase HCl reacting with the adsorbed C 2 H 2 on the catalyst surface [19] , [20] . Figure 3: Catalytic activity of SiC@N-C. ( a ) As a function of reaction temperatures. ( b ) As a function of space velocities. ( c ) At a varying partial pressure of HCl in the feed stream. ( d ) Long-term stability test of SiC@N-C. Reactions were carried out at 200 °C, atmospheric pressure, a space velocity of 0.8 ml g −1 min −1 , HCl/C 2 H 2 =1.15/1 (volume ratio) unless otherwise stated. The selectivity to vinyl chloride is above 98%. Full size image Furthermore, this catalyst exhibits a rather good stability and the acetylene conversion only decreases slightly during a 150 h test at 200 °C, as demonstrated in Fig. 3d . In contrast, the SiC@C sample without N-doping, which was synthesized at the same temperature, yields only a conversion of 24% even though its specific BET (Brunnauer-Emmett-Teller) surface area is higher than that of SiC@N–C ( Supplementary Table 1 ). This highlights the important role of N functionalities in the reaction. Note that no metal species have been used in the synthesis procedure of SiC@N–C. The analysis by Inductively-Coupled Plasma-Atomic Emission Spectrometry (ICP-AES) confirms that the amount of metals in SiC@N–C is negligible ( Supplementary Table 2 ). These results explicitly demonstrate that hydrochlorination of acetylene has been achieved with a N-doped SiC-based carbon catalyst. Active sites for catalytic hydrochlorination of acetylene XPS analysis ( Fig. 2b ) reveals that four types of N species coexist in the SiC@N–C catalyst, that is, pyridinic, pyrrolic, quaternary type N and pyridine oxide. Their structures are schematically displayed in Supplementary Fig. 2 . The pyridinic N bonds with two carbon atoms in the six-membered rings with one p-electron localized in the π system, the pyrrolic type N bonds with two carbon atoms in the five-membered rings, and the quaternary N substitutes one C atom bonding with three C atoms in the six-membered rings [13] . Deconvolution of the N1s spectrum in Fig. 2b indicates that the content of the pyridinic N species in the surface carbon layer, which is defined as the ratio of pyridinic N atom to the sum of surface N, C and O atoms, is 3.0%, pyrrolic N 2.8%, quaternary N 1.2% and very little pyridine oxide. Since these N species differ significantly in their structures, they may function differently in this reaction. However, the coexistence of these different N species in SiC@N–C makes it difficult to assess their respective catalytic roles and not to mention further optimization of the catalyst. Although several methods have been developed for synthesis of N–C materials [21] , [22] , multiple types of N species are often introduced simultaneously. It still remains a challenge to dope carbon materials with a single type of N species. Therefore, we turned to materials dominant with a specific type of N species as model catalysts. C 3 N 4 represents an interesting synthetic carbon material with a total N content as high as 60.9% theoretically and the perfect structure contains only pyridinic and quaternary N, and no pyrrolic N species [23] . We synthesized it following a previously reported method [24] . XPS analysis ( Fig. 4a ) indicates that the content of pyridinic N is 36.5%, quaternary N 8.9% and there is almost no pyrrolic N. As shown in Fig. 4b , this C 3 N 4 catalyst gives only a negligible acetylene conversion at 3.1 ml min −1 g −1 , which implies that the pyridinic and quaternary N may not be the catalytically active sites. Then we investigated the role of pyrrolic N species in the reaction by taking polypyrrole (PPy) as a model catalyst because PPy contains only pyrrolic N species. It is a widely used polymer and can be easily synthesized by polymerization of pyrrole [25] . The obtained PPy has a BET surface area of 10 m 2 g −1 ( Supplementary Table 1 ), which is similar to that of C 3 N 4 . However, PPy yields an acetylene conversion of 26%, which is much higher than C 3 N 4 under the same conditions. Furthermore, the activity of PPy is also approaching that of SiC@N–C although the BET surface area of PPy is significantly lower than that of SiC@N–C. Therefore, pyrrolic N species are most likely responsible for this reaction. 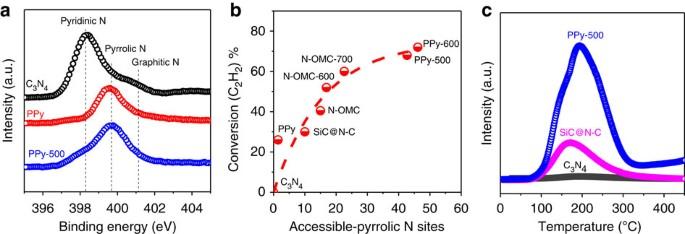Figure 4: Model catalysts containing different N species and their activities in chlorination of acetylene. (a) XPS N1s spectra of C3N4, PPy and PPy-500 (PPy activated with KOH at 500 °C). (b) Acetylene conversion as a function of the accessible-pyrrolic N sites, which are estimated, for comparison, by multiplying the content of pyrrolic N species with the specific BET surface area. Reaction condition: 200 °C, 3.1 ml g−1min−1and HCl/C2H2=1.15/1 (volume ratio). (c) TPD of acetylene on different catalysts. Figure 4: Model catalysts containing different N species and their activities in chlorination of acetylene. ( a ) XPS N1s spectra of C 3 N 4 , PPy and PPy-500 (PPy activated with KOH at 500 °C). ( b ) Acetylene conversion as a function of the accessible-pyrrolic N sites, which are estimated, for comparison, by multiplying the content of pyrrolic N species with the specific BET surface area. Reaction condition: 200 °C, 3.1 ml g −1 min −1 and HCl/C 2 H 2 =1.15/1 (volume ratio). ( c ) TPD of acetylene on different catalysts. Full size image If the N species are assumed to be homogeneously distributed throughout the carbon layer, the low surface area makes it difficult for the reactants to access all the N species. Therefore, we activated PPy using KOH [25] to expose pyrrolic N species as many as possible on the surface. This activation generates pores in the material and the surface area jumps to 535 m 2 g −1 upon treatment at 500 °C (PPy-500). As anticipated, this significantly increases the accessibility of these N sites ( Supplementary Table 1 ). The acetylene conversion rises to 68% under the same reaction conditions although this high temperature activation unfortunately also reduces the content of the pyrrolic N species from 14.7% down to 7.8% ( Supplementary Fig. 3 ), which should have offset the catalytic activity gain to some extent. To further verify the catalytic role of the pyrrolic N species, we compared a series of N–C materials, including PPy activated at 600 °C (PPy-600) and N-doped ordered mesoporous carbon materials, that is, N-OMC, N-OMC-600 and N-OMC-700 (see experimental section for details). As shown in Fig. 4b , the activity increases monotonically with the accessible-pyrrolic N sites irrespective of the varying precursors and N-doping methods. PPy-600 yields a conversion of 72%, equivalent to a vinyl chloride productivity of 2.79 mol kg cat −1 h −1 at 3.1 ml min −1 g −1 ( Supplementary Table 3 ). This lends further support to our proposal that carbon materials doped with pyrrolic N species are active for the reaction. Note that PPy-600 contains only a negligible amount of iron (0.003%) and potassium (0.004%) after thorough washing during synthesis process ( Supplementary Table 2 ). For comparison, we did not remove iron from PPy after oxidation and the resulting Fe-PPy contains around 4.558% iron. It gives a similar activity to PPy, indicating no obvious promoting effect of iron on the hydrochlorination of acetylene. In addition, we used ammonium persulfate ((NH 4 ) 2 S 2 O 8 ) as an oxidant instead of FeCl 3 in the synthesis of PPy. The obtained sample also shows a similar activity (28%) as the previous PPy catalyst under the same conditions, which further demonstrates that iron is not essential for this process. Similarly, if potassium was not removed from PPy after activation at 600 °C, the sample contains around 3.550% potassium, coded as K-PPy-600. This K-PPy-600 gives a conversion of 27%, in contrast to 72% for PPy-600, suggesting a retarding effect of potassium on the hydrochlorination of acetylene. Therefore, the high activity of PPy-600 cannot be primarily attributed to possible iron and potassium residues. Although the effect of the trace potassium is yet to be explored in more detail, it is clear that N species particularly pyrrolic N in carbon play more crucial roles in acetylene hydrochlorination. Temperature-programmed desorption (TPD) is an effective technique providing direct comparison of the adsorption and activation of reactants on different catalysts. The desorption temperature in the TPD profiles reflects the binding strength of the adsorbed species with the catalyst surface and the peak area correlates with the amount of adsorbed species. Figure 4c indicates that there is a considerable amount of acetylene adsorbing on SiC@N–C and PPy-500. The desorption covers the temperature range of 100–300 °C for both samples, which is generally assigned to chemisorbed species, validating the capability of SiC@N–C and PPy-500 for activating acetylene directly. In contrast, there is negligible adsorption of acetylene on C 3 N 4 , which explains the reason for almost no acetylene conversion detected in the reaction. Furthermore, the adsorption amount of acetylene decreases in the following order: PPy-500>SiC@N–C>C 3 N 4 , which agrees well with the activity sequence displayed in Fig. 4b . Reaction mechanism studied by DFT DFT (density functional theory) calculations were carried out to gain further fundamental understanding on the catalytic roles of pyrrolic N sites and the reaction mechanism. We have considered the typical structures of N-doping in carbon including quaternary, pyridinic and pyrrolic N, as depicted in Fig. 5a and b . The results indicate that acetylene hardly adsorbs on the quaternary (Structure 1) and pyridinic N (structure 2 and 3) sites because of the endothermic nature of the adsorption process ( Fig. 5c ). This supports our experimental observation of negligible adsorption of acetylene in TPD and negligible activity of the C 3 N 4 catalyst, which contains only pyridinic and quaternary N species. In contrast, the adsorption becomes exothermic with E a =−0.07 eV on the carbon atoms bonded with pyrrolic N site in structure 4 and it becomes more facile on structure 5 with E a =−0.58 eV owing to the electronic structures of these sites. The projected density of states in Fig. 5d indicates that both the pyrrolic (structure 5) and pyridinic N (structure 2) induce localized electronic states below the Fermi level on the carbon sites in contrast to the quaternary N in structure 1. This is important for the adsorption of acetylene ( Supplementary Fig. 4 ). Furthermore, the pyrrolic-N-induced electronic state possesses a higher energy level and density, which benefits the adsorption of acetylene. The reaction energy profile on structure 5 ( Fig. 5e ) shows that reaction of gas phase HCl with the adsorbed acetylene is strongly exothermic with an activation barrier of 0.91 eV and the energy barrier for desorption of vinyl chloride is 1.16 eV, which are moderate for a reaction at 200 °C. This suggests that carbon doped with pyrrolic N species could catalyze the hydrochlorination of acetylene. 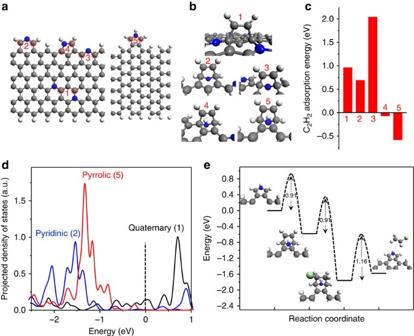Figure 5: DFT calculations on the reaction mechanism. (a) Models with different N species used in DFT calculation, with the blue balls representing N atoms. Structure 1 stands for quaternary N; structure 2 denotes a pyridinic N bonded with two C atoms saturated by H, and structure 3 also pyridinic N but the two neighbour C atoms bonded with another two C; structure 4 represents a pyrrolic N with one C neighbour saturated by H while the other bonded with C and structure 5 also a pyrrolic N but with two C neighbours bonded with H. The C atoms marked with red circles adjacent to N are the adsorption sites for C2H2. (b) The structures with adsorbed C2H2. (c) The corresponding adsorption energies (Ea). (d) The projected density ofpzstates of the C sites for C2H2adsorption. (e) Reaction energy profile of the acetylene hydrochlorination on the pyrrolic structure 5. Figure 5: DFT calculations on the reaction mechanism. ( a ) Models with different N species used in DFT calculation, with the blue balls representing N atoms. Structure 1 stands for quaternary N; structure 2 denotes a pyridinic N bonded with two C atoms saturated by H, and structure 3 also pyridinic N but the two neighbour C atoms bonded with another two C; structure 4 represents a pyrrolic N with one C neighbour saturated by H while the other bonded with C and structure 5 also a pyrrolic N but with two C neighbours bonded with H. The C atoms marked with red circles adjacent to N are the adsorption sites for C 2 H 2 . ( b ) The structures with adsorbed C 2 H 2 . ( c ) The corresponding adsorption energies (E a ). ( d ) The projected density of p z states of the C sites for C 2 H 2 adsorption. ( e ) Reaction energy profile of the acetylene hydrochlorination on the pyrrolic structure 5. Full size image We have also looked into N-free carbon structures because SiC@C exhibits some activity for the hydrochlorination process. The results in Supplementary Figs. 5 and 6 demonstrate that pure carbon may exhibit a limited activity on zigzag edges of graphene sheets. But vinyl chloride is rather difficult to desorb from zigzag edges. This is likely the reason for the much lower activity of SiC@C ( Fig. 3d ) and highlights again the importance of N doping for achieving efficient hydrochlorination of acetylene. We have demonstrated here a nanocomposite N–C deriving from SiC, which catalyzes directly hydrochlorination of acetylene. It exhibits a rather high activity with acetylene conversion reaching 80% and selectivity to vinyl chloride above 98% at a space velocity of 0.8 ml g −1 min −1 and 200 °C. Furthermore, the catalyst remains stable within a test period of 150 h, showing potential to substitute the notoriously toxic mercury chloride for acetylene hydrochlorination. Both experimental and theoretical studies reveal that the carbon atoms bonded with pyrrolic N species are the active sites and the activity increases monotonically with the accessible-pyrrolic N sites. Although no reliable methods are available to determine accurately the number and dispersion of active sites for SiC@N–C, a combination of XPS, TEM and thermogravimetry can be used to estimate the total number of pyrrolic N sites assuming they were distributed homogeneously throughout the carbon layer. Further assuming that the carbon atoms bonded with these pyrrolic N are all active and accessible for acetylene, it leads to a turnover frequency of 1.5 h −1 . Although the pyrrolic materials, such as PPy-600, gives an acetylene conversion twice that of SiC@N–C under the same conditions, they are less suitable for industrial practice because of their powder nature. Still, this points to strategies for further optimization, that is, by increasing the amount of pyrrolic N sites and their accessibility to achieve a higher single pass conversion. The findings also open up an intriguing route to metal-free catalysts for reactions involving other alkynes. Furthermore, such a SiC@N–C composite has other advantages such as being easy to shape, good mechanical strength and heat conductivity and chemical stability, which makes it appealing for applications even in fluidized bed reactors. It would allow operation at a wider range of temperatures and space velocities. With these characteristics, this composite is also promising as a substitution of commercial AC as the catalyst support in a wider range of industrial processes. Catalyst preparation The SiC@N–C catalyst was synthesized by exposing the preshaped SiC granules (20–40 mesh) to a mixture of CCl 4 (Ar saturated with CCl 4 ) and NH 3 with a volume ratio of NH 3 /CCl 4 varying 1/3.7–1/7.4 at 800–1,000 °C [12] . C 3 N 4 was synthesized using SBA-15 as a template following a reported method [24] . Typically, 2 g SBA-15 with a mean pore size of 6 nm was mixed with 5.1 ml cyanamide aqueous solution (50wt.%) and stirred for 5 h. After being dried in air, the material was heated to 550 °C in Ar at a ramp of 1.8 °C min −1 and kept at the same temperature for 4 h. It was subsequently treated with excess 10% hydrofluoric acid aqueous solution for 24 h to remove the SBA-15 template. Then it was washed with distilled water, filtered and dried at 110 °C. PPy was synthesized using pyrrole as the precursor [25] . Pyrrole (3.2 ml) was added to 200 ml aqueous FeCl 3 solution (0.5 M). After stirring for 6 h, the mixture was filtered and washed thoroughly with distilled water to remove iron till no precipitation was observed upon addition of NaOH solution to the filtrate. The sample was then dried at 110 °C overnight. PPy-500 and PPy-600 were obtained by reacting PPy with KOH at 500 and 600 °C under Ar, respectively. Subsequently, potassium was removed by washing with aqueous HCl solution (2 M) and abundant water. For comparison, PPy was also synthesized using ammonium persulfate as oxidant [26] . Pyrrole (3 ml) was added into 200 ml aqueous HCl solution (0.1 M) under stirring. Aqueous solution of (NH 4 ) 2 S 2 O 8 was added slowly to the above mixture under stirring in ice water bath. It was further stirred for 4 h to complete the polymerization of pyrrole. Then the mixture was filtered and washed with abundant water till the filtrate was neutral. Nitrogen-doped ordered mesoporous carbon (N-OMC, N%=2.2%) was purchased from Unicarbon Shanghai Environmental Science & Technology Company. More N species were introduced by treatment at 600 and 700 °C in NH 3 , which were designated as N-OMC-600 (N%=3.2%) and N-OMC-700 (N%=4.4%), respectively. Catalytic reaction Hydrochlorination of acetylene was carried out in a fixed-bed quartz tube reactor at atmospheric pressure and 200 °C. Generally 1.2 g SiC@N–C catalyst (20–40 mesh) was used. A premixed C 2 H 2 /HCl stream with a volume ratio of 1/1.15 was used as the feeding unless otherwise stated. The effluent from the reactor was passed through an aqueous NaOH solution to remove HCl before being fed to an online gas chromatograph. The conversion of acetylene ( X acetylene ) was calculated as: X acetylene =( M VC )/( M VC + M r ) × 100%, where M VC represents the moles of vinyl chloride and M r the moles of the remaining acetylene in the effluent. Turnover frequency was estimated at an acetylene conversion of 18% under 6.2 ml min −1 g −1 . The carbon mass balance was checked during a steady state reaction using CH 4 (5% vol) as the internal standard by comparing the initial carbon moles of acetylene entering the reactor with the total C moles of the unreacted acetylene and vinyl chloride in the effluent. The results show that the carbon mass balance is above 98%. Characterization XPS was carried out on a VG ESCALAB MK2 spectroscope with Al Kα x-rays as the excitation source at 12.5 kV and power of 250 W. The binding energies were calibrated by the contaminant carbon (C1s 284.6 eV). BET surface area was measured by nitrogen physisorption at 77 K on a Micromeretics ASAP 2400 apparatus. Aberration-corrected HRTEM was carried out on an FEI Titan 80–300 with an acceleration voltage of 300 kV. Inductively-coupled plasma atomic emission spectroscopy was carried out at SHIMADZU ICPS-8100. Temperature-programmed desorption The samples were first swept in He before exposure to acetylene (40 ml min −1 ) for 2 h at room temperature. Then it was swept in a flowing He stream (40 ml min −1 ) again until a stable baseline had been obtained. Subsequently, the catalyst was heated to 900 °C at a rate of 10 °C min −1 and the effluent was monitored by an online mass spectrometer (Quadrupole mass spectrometer, Balzers OmniStar 300). The signal of m/e=26 was taken for acetylene. DFT calculations The Vienna Ab-initio Simulation Package (VASP) was used with the projector-augmented wave method and a cutoff energy of 400 eV [27] . The generalized gradient approximation method with Perdew–Burke–Ernzerhof functional for the exchange-correlation term were employed [28] . The N-doping carbon nanoribbon models ( Fig. 5a ) were set in rectangular supercells. The vacuum thickness in the direction perpendicular and parallel to the ribbon plane was set at 12 and 10 Å, respectively. The nanoribbon with armchair and zigzag edges consists of 6 and 5 benzene rings in width, respectively. A wider ribbon model was also tested, which showed a negligible influence on the results. A 4 × 1 × 1 Monkhorst-Pack k-point sampling was used for all models [29] . Spin-polarization was considered for both edges. The convergence of energy and forces were set to 1 × 10 −4 eV and 0.05 eV/Å, respectively. The transition states were searched using the nudged-elastic band method [30] . How to cite this article : Li, X. et al. Nitrogen-doped carbon materials substituting mercury for catalytic hydrochlorination of acetylene. Nat. Commun. 5:3688 doi: 10.1038/ncomms4688 (2014).